A mutation in the receptor Methoprene-tolerant alters juvenile hormone response in insects and crustaceans Juvenile hormone is an essential regulator of major developmental and life history events in arthropods. Most of the insects use juvenile hormone III as the innate juvenile hormone ligand. By contrast, crustaceans use methyl farnesoate. Despite this difference that is tied to their deep evolutionary divergence, the process of this ligand transition is unknown. Here we show that a single amino-acid substitution in the receptor Methoprene-tolerant has an important role during evolution of the arthropod juvenile hormone pathway. Microcrustacea Daphnia pulex and D. magna share a juvenile hormone signal transduction pathway with insects, involving Methoprene-tolerant and steroid receptor coactivator proteins that form a heterodimer in response to various juvenoids. Juvenile hormone-binding pockets of the orthologous genes differ by only two amino acids, yet a single substitution within Daphnia Met enhances the receptor’s responsiveness to juvenile hormone III. These results indicate that this mutation within an ancestral insect lineage contributed to the evolution of a juvenile hormone III receptor system. Juvenile hormones (JHs) are acyclic sesquiterpenoid hormones that regulate important physiological and developmental processes among arthropods, including metamorphosis, moulting, growth, reproduction, sex and caste determination [1] , [2] , [3] , [4] , [5] , [6] , [7] . As exposure of JHs to animals can easily deflect developmental pathways, JHs are well studied in crustaceans for aquaculture [8] , [9] , [10] and in insects for agricultural pest control [11] , [12] . Crustaceans mainly use methyl farnesoate (MF) as the innate JH ligand [13] whereas insects use an epoxide form of MF called JH III (JH III), which is catalysed by the MF epoxidase, CYP15A1 (ref. 14 ). Therefore, MF is the precursor form of active JH in insects [15] , [16] , [17] . However, little is known about their receptor systems and how they evolved. Freshwater microcrustaceans Daphnia pulex and D. magna show striking JH-mediated polyphenisms such as environmental sex determination, induction of haemoglobin in response to reduced oxygen availability in aquatic habitats and inducible morphological defenses against predators signalled by kairomones [8] , [9] , [10] , [18] , [19] , [20] , [21] . In particular, the relationship between environmental sex determination and JH has been well studied over the last decade [8] , [9] , [10] , [22] . Most Daphnia species usually produce female offspring by parthenogenesis; however, once environmental conditions become barren, such as starvation or crowding, they produce male offspring and sexual reproduction occurs [23] . Male production is also induced by topical application of JH and JH analogues independent of environmental condition [8] , [9] , [10] , suggesting that JH is a key endocrine factor for sex determination working downstream of environmental stimuli in Daphnia . 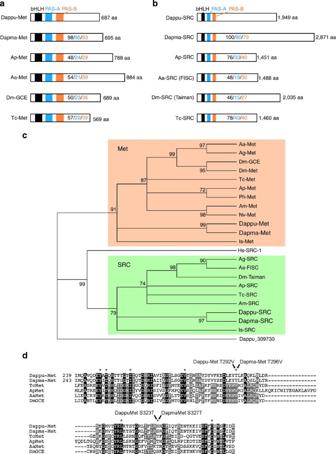Figure 1: Met and SRC in twoDaphniaspecies. (a,b) Met and SRC in twoDaphniaspecies,D. pulex(Dappu) andD. magna(Dapma), and homologues in insect species. BothDaphniaMet (a) and SRC (b) contain bHLH domain and PAS (PAS-A and PAS-B) domain in their sequences. Values in each sequence indicate percentage identity of amino-acid sequences of bHLH (black), PAS-A (blue) and PAS-B (orange) domain with those ofD. pulex. Characteristic SRC family motifs LXXLL and glutamine-rich (Q-rich) regions were identified within the central and C-terminal regions of both Dappu-SRC and Dapma-SRC39. (c) Maximum Likelihood tree based on the amino-acid sequences of Met and SRC suggested thatDaphniaMet and SRC were orthologs of insect Met and SRC, respectively. Dappu_309730 is another protein with bHLH–PAS domain found in the genome database ofD. pulex. Strongly supported nodes (>70%) are labelled with the percentage of bootstrap 1,000 replications. (d) Multiple alignment of PAS-B domain inDaphniaand insect Met. Asterisks indicate eight amino acids involved with JH III binding inTriboliumMet24. In this study, two amino acids indicated by arrows were mutated to the corresponding amino acids used in insects. Species abbreviations and accession codes are as follows:Aedes aegypti(Aa) Met (XP_001660262.1) and SRC (FISC) (ABE99837.2);Anopheles gambiae(Ag) Met (XP_316059.4) and SRC (XP_001689140.1);Apis mellifera(Am) Met (XP_395005.4) and SRC (XP_394114.4);Acyrthocyphon pisum(Ap) Met (XP_003246905.1) and SRC (XP_001944363.2);D. magna(Dapma) Met (AB698069) and SRC (AB698070);D. pulex(Dappu) Met (AB698067) and SRC (AB698068);D. melanogaster(Dm) Met (NP_511126.2), GCE (NP_511160.2) and SRC (Taiman) (AAG16637.1);Homo sapiens(Hs) SRC-1 (AAB50242.1);Ixodes scapularis(Is) Met (XP_002410323.1) and SRC (XP_002402360.1);Nasonia vitripennis(Nv) Met (XP_001606775.2);Pediculus humanus(Ph) Met (XP_002430841.1);Tribolium castaneum(Tc) Met (EFA00995.1) and SRC (EFA04027.1). aa, amino acid. To date, several chemicals, including MF, JH III and four artificially synthesized juvenoids used in this study (that is, fenoxycarb, pyriproxyfen, methoprene and epofenonane), have been shown to be able to induce male daphniids with various concentration ranges [10] , [22] ( Table 1 ). Although receptors of JH are still unknown in any of the crustacean species, basic information obtained from these ecotoxicological studies is helpful in understanding crustacean JH pathway. There is every possibility that the difference in the capacity to induce male, shown by these chemicals, reflects ligand selectivity of JH receptor systems of Daphnia directly. Table 1 EC 50 of transcriptional activation via heterodimerization between SRC and Met (mutant) used in this study. Full size table Methoprene-tolerant (Met) and steroid receptor coactivator (SRC) are proteins that belong to the basic helix–loop–helix (bHLH)–Per–Arnt–Sim (PAS) family of transcription factors. Both have important roles in the JH reception and downstream transcriptional activation [24] , [25] , [26] . Met is regarded as a leading candidate for the JH receptor in insect studies [27] , [28] , [29] . SRC—whose name is from the mammalian homologue SRC-1 with orthologs named FISC and Taiman in Aedes and Drosophila species—is also involved in the reception and signal transduction of JH [24] , [25] , [26] . Although Met exists as a homodimer (or heterodimer with the Drosophila -specific paralog, germ cell-expressed (GCE)) in the absence of JH [30] , the homodimer is remodelled to form a heterodimer with SRC followed by transcriptional activation of downstream elements upon JH binding to the carboxy-terminal PAS domain (PAS-B) of Met [24] , [25] , [26] . To understand the molecular underpinnings of the JH reception system in daphniids and ligand transition that likely occurred when hexapods evolved from their pancrustacean ancestor [31] , we tested the JH sensitivity of Met and SRC in two crustacean species, D. pulex and D. magna . As a result, Daphnia Met and SRC showed capability to respond to various juvenoid in different dose ranges, respectively. Moreover, we demonstrate that a single amino-acid substitution within Daphnia Met enhances the receptor’s responsiveness to JH III, suggesting that this mutation contributed to the evolution of a JH III receptor system. Cloning and characterization of Daphnia Met and SRC We cloned and characterized the full-length sequences of Met and SRC genes from two Daphnia species, designated as Dappu-Met and Dappu-SRC for D. pulex , and Dapma-Met and Dapma-SRC for D. magna (accession numbers: AB698067–AB698070). Pairwise sequence identities of bHLH, PAS-A and PAS-B domains between Daphnia and selected insect species range from 15% to 78% ( Fig. 1a–c ). Six of eight polymorphic amino-acid residues within PAS-B domain forming JH-binding pockets are conserved in Met of both Daphnia species [25] ( Fig. 1d ). At the other two sites, valine in insects is substituted for threonine in Daphnia , and threonine in insects is substituted by serine ( Fig. 1d ). We hypothesize that one or both amino-acid substitutions cause differences in ligand specificity of Met between crustaceans and insects. Both genes are required for development; transcriptional knockdown of Dapma-Met or Dapma-SRC result in embryonic death ( Fig. 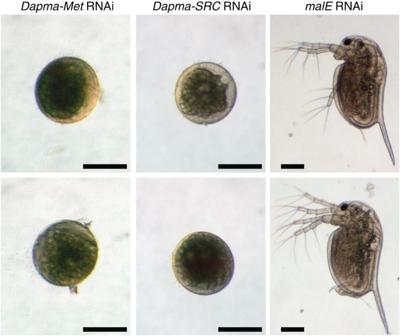Figure 2: Phenotypes of RNA interference (RNAi) targeting of theDapma-MetandDapma-SRC. Development ofDapma-MetorDapma-SRCdsRNA-injected embryos was aborted at 20–30 h after oviposition.E. coli malEdsRNA-injected embryos grew into the first instar juveniles at 80 h after oviposition. Scale bars, 200 μm. 2 and Table 2 ). Figure 1: Met and SRC in two Daphnia species. ( a , b ) Met and SRC in two Daphnia species, D. pulex (Dappu) and D. magna (Dapma), and homologues in insect species. Both Daphnia Met ( a ) and SRC ( b ) contain bHLH domain and PAS (PAS-A and PAS-B) domain in their sequences. Values in each sequence indicate percentage identity of amino-acid sequences of bHLH (black), PAS-A (blue) and PAS-B (orange) domain with those of D. pulex . Characteristic SRC family motifs LXXLL and glutamine-rich (Q-rich) regions were identified within the central and C-terminal regions of both Dappu-SRC and Dapma-SRC [39] . ( c ) Maximum Likelihood tree based on the amino-acid sequences of Met and SRC suggested that Daphnia Met and SRC were orthologs of insect Met and SRC, respectively. Dappu_309730 is another protein with bHLH–PAS domain found in the genome database of D. pulex . Strongly supported nodes (>70%) are labelled with the percentage of bootstrap 1,000 replications. ( d ) Multiple alignment of PAS-B domain in Daphnia and insect Met. Asterisks indicate eight amino acids involved with JH III binding in Tribolium Met [24] . In this study, two amino acids indicated by arrows were mutated to the corresponding amino acids used in insects. Species abbreviations and accession codes are as follows: Aedes aegypti (Aa) Met (XP_001660262.1) and SRC (FISC) (ABE99837.2); Anopheles gambiae (Ag) Met (XP_316059.4) and SRC (XP_001689140.1); Apis mellifera (Am) Met (XP_395005.4) and SRC (XP_394114.4); Acyrthocyphon pisum (Ap) Met (XP_003246905.1) and SRC (XP_001944363.2); D. magna (Dapma) Met (AB698069) and SRC (AB698070); D. pulex (Dappu) Met (AB698067) and SRC (AB698068); D. melanogaster (Dm) Met (NP_511126.2), GCE (NP_511160.2) and SRC (Taiman) (AAG16637.1); Homo sapiens (Hs) SRC-1 (AAB50242.1); Ixodes scapularis (Is) Met (XP_002410323.1) and SRC (XP_002402360.1); Nasonia vitripennis (Nv) Met (XP_001606775.2); Pediculus humanus (Ph) Met (XP_002430841.1); Tribolium castaneum (Tc) Met (EFA00995.1) and SRC (EFA04027.1). aa, amino acid. Full size image Figure 2: Phenotypes of RNA interference (RNAi) targeting of the Dapma-Met and Dapma-SRC . Development of Dapma-Met or Dapma-SRC dsRNA-injected embryos was aborted at 20–30 h after oviposition. E. coli malE dsRNA-injected embryos grew into the first instar juveniles at 80 h after oviposition. Scale bars, 200 μm. Full size image Table 2 Summary of the result of RNAi transcriptional knockdown experiments. Full size table JH-dependent heterodimerization of Daphnia Met and SRC We tested juvenoid-dependent Met–SRC protein interactions in Daphnia by two-hybrid luciferase assay [25] , [32] (see Methods). MF (JH in crustaceans), JH III (JH in insects) and four artificially synthesized juvenoids (fenoxycarb, pyriproxyfen, methoprene and epofenonane) were used for this study. As described above, all these chemicals induce male offspring development in Daphnia [10] , [22] ( Table 1 ). We detected concentration-dependent luciferase activation from the heterodimerization of Met with SRC by all juvenoid treatments, except for epofenonane ( Fig. 3a ). Although the effective dose responses to the juvenoids vary for both species, parallel responses are observed suggesting that the Met–SRC complex functions as a JH receptor in Daphnia species, as in insects [24] , [25] , [26] . In addition, the effect of MF on heterodimerization is nearly tenfold greater than that of JH III, which is consistent with the knowledge that crustaceans use MF as an active form of JH ( Fig. 3a and Table 1 ), not JH III. Dappu-Met and Dapma-Met were also swapped in combination with Dapma-SRC and Dappu-SRC for each of the treatments. These swapped pairs also exhibited juvenoid-dependent dimerization (Fig. 5), yet combinations of both Met–Met and SRC–SRC did not show juvenoid-dependent responses (Fig. 5), thus further confirming that the Met and SRC protein complex functions as a JH receptor in daphniids. 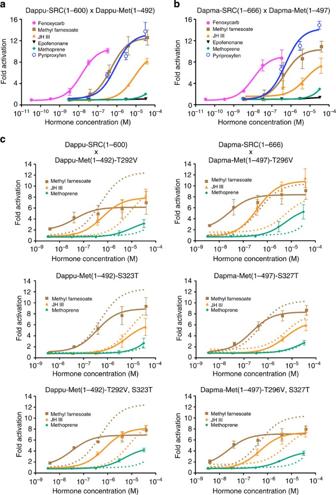Figure 3: Transcriptional activation via heterodimerization betweenDaphniaMet and SRC exposed to various juvenoids. (a) Concentration–response profile for SRC(1–600) and wild-type Met(1–492) ofD. pulex. (b) Concentration–response profile for SRC(1–666) and wild-type Met(1–497) ofD. magna. (c) Concentration–response profile for SRC and mutant Met. Vertical axis indicates fold activation, which is the luciferase activity normalized by solvent control (0.1% ethanol) of each experiment. Dotted lines indicate profiles of wild types. Each point represents the mean of triplicate determinations, and vertical bars represent the mean±s.d. Figure 3: Transcriptional activation via heterodimerization between Daphnia Met and SRC exposed to various juvenoids. ( a ) Concentration–response profile for SRC(1–600) and wild-type Met(1–492) of D. pulex . ( b ) Concentration–response profile for SRC(1–666) and wild-type Met(1–497) of D. magna . ( c ) Concentration–response profile for SRC and mutant Met. Vertical axis indicates fold activation, which is the luciferase activity normalized by solvent control (0.1% ethanol) of each experiment. Dotted lines indicate profiles of wild types. Each point represents the mean of triplicate determinations, and vertical bars represent the mean±s.d. Full size image Transition of JH ligand sensitivity Finally, we tested our hypothesis that the threonine → valine and/or serine → threonine amino-acid substitutions in Met cause different ligand specificities of the receptor between crustaceans and insects, by measuring ligand-dependent heterodimerization using mutant Daphnia Met ( Fig. 1d ) that have amino acids T292V in Dappu-Met and T296V in Dapma-Met exchanged with Val-297 of Tribolium Met, and have amino acids S323T in Dappu-Met and S327T in Dapma-Met exchanged with Thr-330, also of the Tribolium gene ( Fig. 1d ). MF, JH III and methoprene treatments were used in this last experiment. For both Daphnia Met genes, the Val-297 mutation significantly increases the receptor sensitivity to JH III ( Fig. 3c and Table 1 ). By contrast, mutations S323T and S327T did not alter ligand sensitivity ( Fig. 3c and Table 1 ). Although there are a lot of reports about the effect of juvenoids on environmental sex determination in daphniids [8] , [9] , [10] , [22] , their JH receptor molecules have been unclear to date. Here, we cloned Met and SRC from two Daphnia species, and demonstrated that Met and SRC proteins form heterodimer only in the presence of juvenoids, suggesting that these molecules act as a JH receptor in crustaceans as in insects [24] , [25] , [26] . Moreover, ligand selectivity that was estimated from the half maximal effective concentration (EC 50 ) values for heterodimerization was generally in accord with previous data for inducing male offspring development when testing six juvenoids (EC 50 values: fenoxycarb<MF<JH III<methoprene; Table 1 and Fig. 4 ) [10] , [22] . Although EC 50 values of pyriproxyfen and epofenonane were not consistent between these two different experiments, the observed difference between the effective ranges for male offspring induction in the two species is likely caused by ligand selectivity of Met (or the Met–SRC complex) for juvenoids. Epofenonane is the only tested compound that does not induce heterodimerization, despite its effect at inducing male offspring development ( Fig. 3a and Table 1 ). For most juvenoids, male induction is also associated with a great reduction of the number of offspring. In contrast, epofenonane can also induce male production with only a slight change in brood size [10] , [22] . It is therefore likely that epofenonane induces male production by a different mechanism from the other juvenoids and their synthetic derivatives, which might not involve Met and SRC. On the other hand, in several insects, juvenoids lead to dissociation of Met–Met homodimer [25] , [30] , yet combinations of two Met plasmids in daphniids indicated neither homodimerization nor juvenoid-dependent responses ( Fig. 5 ), thus further confirming that the Met and SRC protein complex functions as a JH receptor in daphniids. 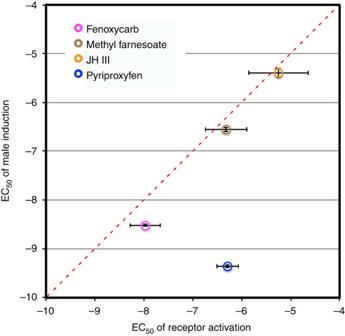Figure 4: Logarithmic relationships between EC50of receptor activation and juvenoid induction of males inD. magna. Error bars indicate 95% confidence intervals. Dotted line indicates log ratio (1). EC50values of male induction are based on the data of previous studies (Tatarazakoet al.10and Odaet al.22(see Table 1)). Figure 4: Logarithmic relationships between EC 50 of receptor activation and juvenoid induction of males in D. magna. Error bars indicate 95% confidence intervals. Dotted line indicates log ratio (1). EC 50 values of male induction are based on the data of previous studies (Tatarazako et al. [10] and Oda et al. [22] (see Table 1)). 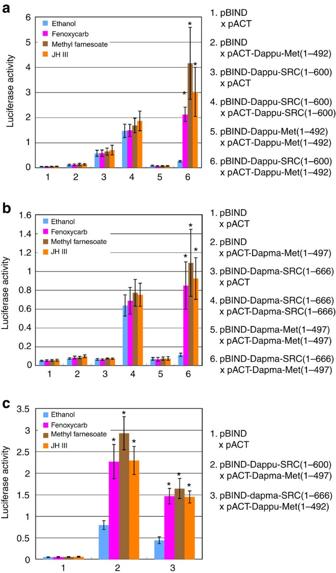Figure 5: Transcriptional activations with various vector combinations. (a) Response profile ofD. pulex. (b) Response profile ofD. magna. (c) Response profile for SRC and Met from differentDaphniaspecies compared with each other. Vertical axis indicates luciferase activities. Each point represents the mean of triplicate determinations, and vertical bars represent the mean±s.d. Asterisks indicate significant differences (P<0.05,t-test) from ethanol treatment of each vector combination. Concentrations of juvenoid (M) used in this experiment are as follows: fenoxycarb (3.32E−08), methyl farnesoate (3.99E−06) and JH III (3.75E−05). Full size image Figure 5: Transcriptional activations with various vector combinations. ( a ) Response profile of D. pulex . ( b ) Response profile of D. magna . ( c ) Response profile for SRC and Met from different Daphnia species compared with each other. Vertical axis indicates luciferase activities. Each point represents the mean of triplicate determinations, and vertical bars represent the mean±s.d. Asterisks indicate significant differences ( P <0.05, t -test) from ethanol treatment of each vector combination. Concentrations of juvenoid (M) used in this experiment are as follows: fenoxycarb (3.32E−08), methyl farnesoate (3.99E−06) and JH III (3.75E−05). Full size image For both Daphnia Met genes, the Val-297 mutation significantly increases the receptor sensitivity to JH III ( Fig. 3c and Table 1 ), suggesting that amino-acid substitution to valine at this site had contributed to the transition of JH ligand during insect evolution. Furthermore, this amino-acid substitution to valine is thought to be involved in reception of methoprene, to which daphniids show lower sensitivity than insects, consistent with a previous report demonstrating that a single amino-acid mutation at Val-297 in Tribolium Met inhibited binding of methoprene to Met [24] . This mutation, however, also increases sensitivity to MF ( Fig. 3c and Table 1 ). Several studies report detectable amounts of MF in insect haemolymph, together with other juvenoids [7] , [33] , [34] . Further studies are required to determine whether both JH III and MF target the same insect receptor. By contrast, mutations S323T and S327T did not alter ligand sensitivity ( Fig. 3c and Table 1 ), possibly because both serine and threonine have similar biochemical characteristics [35] . Given that a similar substitution to threonine can also be found within the Drosophila melanogaster GCE ( Fig. 1d ), it is thought to be a less functional polymorphism during the evolution of JH receptor. In summary, present study strongly suggests that the Met–SRC complex operates as a JH receptor in daphniids as well as insects, but their ligand sensitivities are somewhat different from each other. It can be a reason why each juvenoid shows so varied effects and toxicity depending on animal species and taxa. Moreover, a single amino-acid substitution is revealed important during evolution of the arthropod JH pathway, by comparative functional genetic studies using a branchiopod crustacean model species. This knowledge, coupled with the identification of a JH-synthesizing organ and isolation of JH-responsive elements interacting with Met–SRC complex, is expected to provide a more unified mechanistic understanding of the development and environmentally induced phenotypic plasticity across Arthropoda. Animals The D. pulex and D. magna clones used in the experiments were provided by the National Institute for Environmental Studies (NIES), Tsukuba, Japan. The clones were reared in the laboratory at 20 °C in aged tap water and fed unicellular green algae (Chlorella Industry Co. Ltd, Fukuoka, Japan) over generations in 1 l beakers in a temperature- and photocycle-controlled incubator (20 °C, 16-h light/8-h dark). Cloning of Met and SRC Amino-acid sequences of insect Met and SRC homologues were obtained using euGene’s Arthropod genomes ( http://insects.eugenes.org/arthropods/ ), and aligned by the ClustalX program [36] using default options. Based on the aligned sequences, conserved regions were identified and used to perform TBLASTN searches against the wFleaBase ( http://wfleabase.org/ ) to identify D. pulex gene models. PCR primers for cloning were designed based on sequences of these gene models. Total RNA was extracted from ~20 adult D. pulex and D. magna using an SV Total RNA Isolation System (Promega, Madison, WI) and converted to complementary DNA using Superscript III and random primers (Life Technologies, Carlsbad, CA) according to the manufacturer’s protocol. Partial sequences of Met and SRC were obtained by PCR amplification, and full-length cDNAs were obtained by GeneRacer Kit (Life Technologies). Domain and motif searches were performed with obtained sequences using the European Bioinformatics Institute (EBI) InterPro database ( http://www.ebi.ac.uk/Tools/InterProScan/ ). Phylogenetic analysis The amino-acid sequences were aligned by the MEGA5 software using default options [37] . The Maximum Likelihood tree was constructed from this alignment using a 1,000 replicate bootstrap analysis, along with complete deletion options. RNA interference Knockdown of Dapma-Met and Dapma-SRC was performed using RNA interference technique according to our previous study [38] . Escherichia coli malE gene was used as a negative control. Double-stranded RNA (dsRNA) was synthesized using the MEGAscript RNAi Kit (Life Technologies). Eggs were obtained from D. magna at 2 weeks of age just after ovulation and placed in ice-cold M4 medium containing 80 mM sucrose (M4-sucrose). The synthesized dsRNA (2 mg ml −1 ) was mixed with 2 mM Chromeo 494 fluorescent dye (Active Motif Chromeon GmbH, Tegernheim, Germany), which was used as a visible marker for injection. Mixture containing 1 mg ml −1 dsRNA was injected to eggs under a microscope. Then, injected eggs were transferred into new Petri dishes and incubated at 20 °C. Construction of the reporter system We used a two-hybrid system to detect heterodimerization of Met and SRC. Chinese hamster ovary cells were transfected according to the instructions [32] with slight modifications. Dappu-Met(1–492) and Dapma-Met(1–497) were cloned into pBIND, and Dappu-SRC(1–600) and Dappu-SRC(1–666) (bHLH–PAS domain) were cloned into pACT (Promega). For transfections, Chinese hamster ovary cells were grown in 1:1 mixture of Dulbecco’s Modified Eagle’s Medium and Ham’s F-12 containing 10% fetal bovine serum, and incubated at 37 °C in a 5% CO 2 atmosphere. The day before transfection, cells were transferred to a 24-well plate. The transfection was performed using FuGENE HD (Promega), according to the manufacturer’s protocols. Each well received 0.05 mg pBIND, 0.05 mg pACT and 0.2 mg pG5luc, which has luciferase gene under the control of GAL4-binding site. All juvenoids were dissolved in ethanol and added to the medium after 24 h, and cells were harvested after 48 h. Reporter activities were measured using the Dual-Luciferase Assay kit (Promega), according to the manufacturer’s protocols. All transfections were performed at least three times, employing triplicate sample points in each experiment. The values shown are mean±s.d. from three separate experiments, and dose–response data and EC 50 were analysed using GraphPad Prism (Graph Pad Software, Inc., San Diego, CA). How to cite this article: Miyakawa, H. et al. A mutation in the receptor Methoprene-tolerant alters juvenile hormone response in insects and crustaceans. Nat. Commun. 4:1856 doi: 10.1038/ncomms2868 (2013).